A new raptorial dinosaur with exceptionally long feathering provides insights into dromaeosaurid flight performance Microraptorines are a group of predatory dromaeosaurid theropod dinosaurs with aerodynamic capacity. These close relatives of birds are essential for testing hypotheses explaining the origin and early evolution of avian flight. Here we describe a new ‘four-winged’ microraptorine, Changyuraptor yangi , from the Early Cretaceous Jehol Biota of China. With tail feathers that are nearly 30 cm long, roughly 30% the length of the skeleton, the new fossil possesses the longest known feathers for any non-avian dinosaur. Furthermore, it is the largest theropod with long, pennaceous feathers attached to the lower hind limbs (that is, ‘hindwings’). The lengthy feathered tail of the new fossil provides insight into the flight performance of microraptorines and how they may have maintained aerial competency at larger body sizes. We demonstrate how the low-aspect-ratio tail of the new fossil would have acted as a pitch control structure reducing descent speed and thus playing a key role in landing. The Late Jurassic–Early Cretaceous deposits of northeastern China are renowned for their exceptional fossil preservation and for yielding a variety of feathered non-avian dinosaurs that have cemented the notion that birds evolved from theropod dinosaurs [1] , [2] . Paramount among these is a variety of small ‘four-winged’ paravian theropods (that is, Microraptor zhaoianus , Pedopenna daohugouensis , Anchiornis huxleyi and Xiaotingia zhengi ) that, in addition to having well-developed wings, had long pennaceous feathers attached to both the tibia and the metatarsus (‘hindwings’) [3] , [4] , [5] , [6] . Recently, these fossils have been drawn to the centre of discussions about the origin of avian flight, but their specific role within this century-old debate still hinges upon a better understanding of their anatomy, aerodynamic capabilities and phylogenetic placement. We report the discovery of the largest known ‘hind-wing’ paravian (HG B016), a microraptorine dromaeosaurid with exceptionally long tail feathers forming an aerodynamic surface of low aspect ratio. Our study indicates that the feathered tail of this new dinosaur was instrumental for decreasing descent speed and assuring a safe landing. Systematic palaeontology Dinosauria, Owen, 1842 Saurischia, Seeley, 1888 Theropoda, Marsh, 1881 Paraves, Sereno, 1997 Dromaeosauridae, Matthew and Brown, 1922 Changyuraptor yangi gen. et sp. nov. Holotype HG B016 (Paleontological Center, Bohai University, Jinzhou City, China) ( Fig. 1 ; Supplementary Fig. 1 ), a complete articulated specimen with extensive feathering. HG B016 constitutes an adult individual based on skeletochronology and it is split in two slabs. 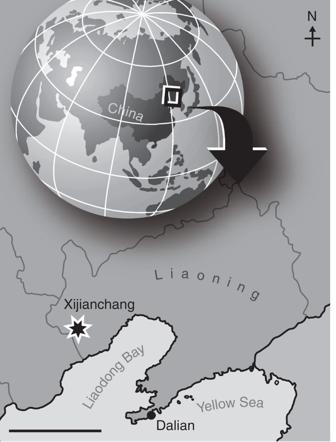Figure 1: Map of Liaoning Province in northeastern China. Xijianchang, the locality where HG B016 was found is indicated by a star. Scale bar, 200 km. Figure 1: Map of Liaoning Province in northeastern China. Xijianchang, the locality where HG B016 was found is indicated by a star. Scale bar, 200 km. Full size image Etymology ‘Changyu’ means ‘long feather’ in Chinese and ‘raptor’ refers to the predatory habits inferred for the holotype. The species name honours Professor Yang Yandong, Chairman of the Bohai University (Liaoning Province, China), who provided the financial support to acquire the specimen. Locality Xijianchang, Jianchang County, Liaoning Province (China); Yixian Formation, Early Cretaceous. Diagnosis A microraptorine dromaeosaurid theropod characterized by having the unique combination of traits: furcula more robust than that of Sinornithosaurus millenii and much larger than that of Tianyuraptor ostromi ; forelimb proportionally much longer when compared with hindlimb than in other microraptorines; humerus much longer (>20% longer) than ulna as opposed to Microraptor zhaoianus , in which these bones are more comparable in length; metacarpal I proportionally shorter than in Sinornithosaurus millenii (1/4–1/5 versus 1/3); well-developed semi-lunate carpal covering all of proximal ends of metacarpals I and II as opposed to the small semi-lunate carpal that covers about half of the base of metacarpals I and II in most other microraptorines; manual ungual phalanx of digit II is the largest, followed by that of digits I andt III, as opposed to Graciliraptor lujiatunensis in which the ungual of manual digit I is very small, and Sinornithosaurus millenii and Microraptor zhaoianus in which the unguals of manual digits I and II are comparable in size; ischium shorter than in Microraptor zhaoianus ; midshaft of metatarsal IV significantly broader than that of metatarsal III or metatarsal II, as opposed to G. lujiatunensis in which metatarsal IV is the narrowest; mid-caudals roughly twice the length of dorsals as in Sinornithosaurus millenii as opposed to long caudal vertebrae in Microraptor zhaoianus ; fewer caudal vertebrae (22 vertebrae) than Microraptor zhaoianus (25–26 vertebrae) and Tianyuraptor ostromi (28 vertebrae); rectrices significantly longer than in other microraptorines. Description The new fossil, HG B016, comes from the Aptian (~125 mya) Yixian Formation [7] , [8] at Xijianchang, Liaoning Province, China ( Fig. 1 ). HG B016, the only known ‘four-winged’ dromaeosaurid from the Yixian Formation, is preserved in two slabs (A and B) and is largely exposed in lateral view. The new specimen has a total length (tip of rostrum to end of tail feathering) of ~132 cm ( Fig. 2 ) ( Table 1 ). Its skull is poorly preserved beyond its dentition. It bears four premaxillary teeth, at least seven teeth in the maxilla and 14–15 in the dentary. The teeth are recurved with serrations on both mesial and distal margins that, as in dromaeosaurids, are larger along the distal margin [9] ( Fig. 3 ). Unlike Microraptor zhaoianus [3] but similar to Graciliraptor lujiatunensis [10] , the tooth crowns of HG B016 are not separated from their roots by a constricted ‘waist’. The boomerang-shaped furcula is large, with broad rami and a ~100° interclavicular angle, a common morphology among basal paravians [11] . The forelimb is long with respect to the hindlimb; its total length (including digit II) is 96% of the hindlimb (including digit III). This ratio contrasts with the shorter forelimbs of other Jehol dromaeosaurids (53% in Tianyuraptor ostromi , 75% in Sinornithosaurus millenii and 89% in Microraptor zhaoianus ) [3] , [12] , [13] . The humerus is significantly longer than the radius-ulna (>20%), as opposed to Sinornithosaurus millenii and Microraptor zhaoianus in which these elements are subequal [3] , [12] . Metacarpal I is approximately one-fourth the length of metacarpal II, similar to Microraptor zhaoianus and shorter than in Sinornithosaurus millenii , in which this ratio is approximately one-third [14] . The recurved manual claws of HG B016 bear strong flexor tubercles and preserve horny sheaths. Manual digit II carries the largest claw, followed by that of digit I and digit III. The rib cage is composed of at least 10 thoracic ribs of which the first through sixth preserve portions of their uncinate processes, unfused to the rib. There appears to be 13 rows of gastralia. 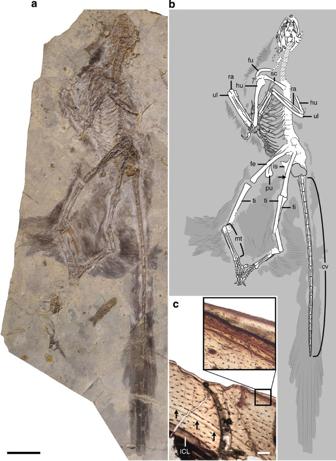Figure 2: Photograph and interpretive drawing of HG B016. Photograph of slab A (a) Composite line drawing of HG B016 based on slabs A and B (b; scale same as ina), and histological thin-section of the midshaft of the right femur of slab B (c). cv, caudal vertebrae; fe, femur; fi, fibula; fu, furcula; hu, humerus; ICL, inner circumferential layer; is, ischium; mt, metatarsals; pu, pubis; ra, radius; sc, scapula; ti, tibia, ul, ulna. Black arrow inbpoints at the location of the histological sample. Inset inchighlights the rest lines visible in the peripheral region of the cortex; the three black arrows incpoint at the earliest visible LAG. Scale bar, 10 cm (a), 200 um (c). Figure 2: Photograph and interpretive drawing of HG B016. Photograph of slab A ( a ) Composite line drawing of HG B016 based on slabs A and B ( b ; scale same as in a ), and histological thin-section of the midshaft of the right femur of slab B ( c ). cv, caudal vertebrae; fe, femur; fi, fibula; fu, furcula; hu, humerus; ICL, inner circumferential layer; is, ischium; mt, metatarsals; pu, pubis; ra, radius; sc, scapula; ti, tibia, ul, ulna. Black arrow in b points at the location of the histological sample. Inset in c highlights the rest lines visible in the peripheral region of the cortex; the three black arrows in c point at the earliest visible LAG. Scale bar, 10 cm ( a ), 200 um ( c ). Full size image Table 1 Selected measurements (in mm) of HG B016 ( Changyuraptor yangi ) and some specimens of the microraptorines Sinornithosaurus haoiana and Microraptor zhaoianus . 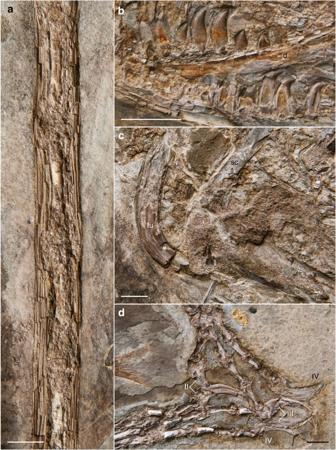Figure 3: Details of the skeleton of slab A of HG B016. (a) Mid portion of the caudal series, (b) dentary teeth, (c) furcula and shoulder girdle and (d) pedal digits. d, dentary; fu, furcula; sc, scapula; II–IV, pedal digits II–IV. Scale bar, 1 cm. Full size table Figure 3: Details of the skeleton of slab A of HG B016. ( a ) Mid portion of the caudal series, ( b ) dentary teeth, ( c ) furcula and shoulder girdle and ( d ) pedal digits. d, dentary; fu, furcula; sc, scapula; II–IV, pedal digits II–IV. Scale bar, 1 cm. Full size image The pelvis is opistopubic. The pubis is more than two-thirds the length of the femur and more than twice the length of the ischium. The distal half of the pubis curves caudally, and its distal end expands to form a spatulate-shape typical of some other Jehol dromaeosaurids. The ischium has a pointed obturator process and a relatively straight distal margin. It is shorter than the ischium of Microraptor zhaoianus and its distal base is proportionally broader. The ischium is most similar to that of Sinornithosaurus millenii , although its concave cranial margin is less excavated. The tibia is slightly longer than the femur. The broad proximal end of the fibula tapers down to a rod-like bone at approximately one-fourth the length of the tibia and it reaches the end of the tibia. The metatarsus is approximately two-thirds the length of the tibia. Metatarsal V is long, straight and rod-like; it exceeds half the length of the metatarsus. Metatarsal III is the longest, followed by metatarsals IV and II. HG B016 shows no evidence of either metatarsal I or its digit, but such an absence may be preservational. Like in Microraptor zhaoianus , the midshaft of metatarsal IV is significantly broader than that of metatarsal III or metatarsal II. Pedal digit III is the longest, followed by digits IV and II. The pedal claws are recurved with slightly bulging flexor tubercles and preserve portions of their horny sheaths. The claw of digit II is the largest, followed by that of digits III and IV. However, digit II lacks the raptorial specializations typical of most other dromaeosaurids (that is, the claw is proportionally smaller and the non-ungual phalanges lack the degree of hyper-extensor capacity of Laurasian eudromaeosaurids) [15] . Surrounding the trochlea of metatarsal IV and between the pedal digits IV and III, there are portions of the tuberculate integument comparable to that reported for Sinornithosaurus millenii [12] . The tail is stiffened by long prezygapophyseal and haemal arch bundles characteristic of most dromaeosaurids [12] , [15] , [16] , [17] , [18] , [19] ( Fig. 3 ). The tail of HG B016 is proportionally shorter than in Tianyuraptor ostromi and Microraptor zhaoianus but longer than in Sinornithosaurus millenii (tail/femur ratio is ~3.8 in HG B016). There are 20 preserved caudal vertebrae with probably no more than the two most proximal vertebrae missing or obstructed by a large concretion ( Fig. 2 ). Thus, a conservative estimate of the caudal count is 22. This is fewer than estimates for other Jehol dromaeosaurids (for example, 28 in Tianyuraptor ostromi , 25–26 in Microraptor zhaoianus ) [17] . The length of the caudal vertebrae increases through the first preserved four vertebrae. Following the preserved 4th caudal, the longest, the vertebral centra remain more or less constant through the preserved 6th caudal before gradually decreasing in length. Unlike Microraptor zhaoianus where the mid-caudals are three to four times the length of the dorsal vertebrae [19] , in HG B016 the mid-caudals are only about two times the length of the dorsal vertebrae making it more similar to the other Yixian dromaeosaurids. The plumage ( Fig. 4 ) is preserved along the ventral portion of the neck and shoulder girdle, dorsal to the pelvis, and along the edge of the forelimbs, hind limbs and tail. Full sets of pennaceous feathers form extensive ‘hindwings’ as in the paravians Microraptor zhaoianus [3] , [20] , [21] , Pedopenna daohugouensis [4] , Anchiornis huxleyi [5] and Xiaotingia zhengi [6] . The hind limbs carry feathers down to the distal end of the metatarsus but there is no feathering attached to the digits (as opposed to Anchiornis zhengi ). The feathers of the ‘hindwings’ are largely overlapping, which prevents determining an exact number and whether they are asymmetric or not. Their lengths cannot be estimated with precision, but some of the feathers projecting from the right ankle are ~135 mm. Long pennaceous feathers are also preserved along most of the length of the tail. These lengthy, symmetrical rectrices project backwards at a slight angle (~20 degrees over most of the tail) from the vertebral axis. They exhibit strong rachises and the vanes remain barbed throughout the length of the feathers. Those projecting from the distal one-fourth of the bony tail are longer and they form a terminal fan composed of at least 8, and perhaps 9, pairs of incrementally longer feathers. The longest feathers of this graduated tail are the central pair of rectrices, with a preserved length of 292.7 mm ( Fig. 4 ). However, the tips of these feathers are missing, indicating that they were even longer. Conservative size estimates of the central rectrices and the tail indicate that these feathers are ~52% of the length of the tail as opposed to 37% in Microraptor zhaoianus [21] . The feathers surrounding the forelimbs are poorly preserved but the shafts of some pennaceous primaries project from the distal end of the left hand. The feathering preserved along the ventral side of the neck and dorsal to the pelvis and base of the tail consists of filamentous appendages similar to those described for Sinornithosaurus millenii [12] , [22] . 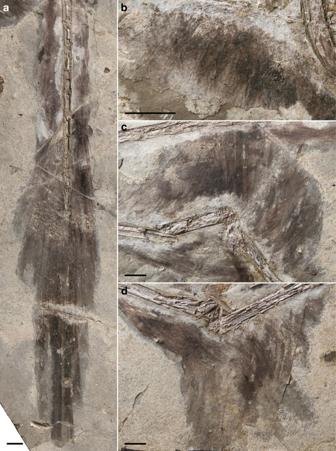Figure 4: Details of the plumage of HG B016 as preserved on slab A. (a) Graduated distal rectrices, (b) feathers surrounding the shoulder girdle, (c) portion of the left hindwing and (d) portion of the right hindwing. Scale bar, 2 cm. Figure 4: Details of the plumage of HG B016 as preserved on slab A. ( a ) Graduated distal rectrices, ( b ) feathers surrounding the shoulder girdle, ( c ) portion of the left hindwing and ( d ) portion of the right hindwing. Scale bar, 2 cm. Full size image Histological analysis of the left femur on slab B ( Fig. 2 ; Supplementary Figs 2, 3 ) reveals that HG B016 had reached adult body size at the time of death. This section shows that the bone wall is ~1 mm in thickness and lacks secondary reconstruction (that is, secondary osteons or erosion cavities). The femoral compact tissue comprised fibro-lamellar bone with mainly longitudinally oriented channels and occasional radial anastomoses. A distinctive line of arrested growth (LAG) interrupts the deposition of the fibro-lamellar bone. A narrow band of lamellar bone tissue, the inner circumferential layer (ICL), lines the medullary cavity. The general nature of the bone tissue suggests that some resorption had preceded the deposition of the ICL. The peripheral region of the bone wall shows a narrow band of tissue with at least three rest lines. The overall histology indicates that the specimen was an adult and at least in its fifth year of postnatal growth when it died. In order to test the phylogenetic placement of HG B016 within paravian theropods, we conducted a cladistic analysis using the data set from Turner et al . [19] The strict consensus of all the most parsimonious trees supports the identification of HG B016 as a Dromaeosauridae ( Fig. 5 ; Supplementary Fig. 4 ) and resolves it within the monophyletic but unresolved Microraptorinae clade ( Fig. 5 ). A monophyletic Dromaeosauridae and Troodontidae are recovered with the avian clade (Aves) as the sister taxon to Deinonychosauria (Dromaeosauridae+Troodontidae). The basal paravian Epidexipteryx hui is the sister taxon to the Aves+Deinonychosauria clade. Relationships among paravians are identical to those found by Turner et al . [19] ( Supplementary Fig. 4 ). A monophyletic but unresolved Microraptorinae clade was recovered and included Hesperonychus elizabethae , Graciliraptor lujiatunensis , Microraptor zhaoianus , Sinornithosaurus millenii and Tianyuraptor ostromi in addition to HG B016. Five unambiguous synapomorphies (character numbers following Turner et al .) support this grouping: a small semi-lunate carpal that covers about half of the base of metacarpals I and II (reversed in Changyuraptor yangi ) (c148.1); metatarsal II proximal shaft constricted and much narrower than either metatarsal II or IV, but still exposed along most of metapodium (subarctometatrsal) (c203.1); lateral face of pubic shaft with a prominent lateral tubercle about halfway down the shaft (c231.1); very elongate extensions of the posterior extensions of the caudal chevrons (c442.1); and combined length of metatarsal I plus phalanx I-1 equal to or less than length of metatarsal II (c444.1). 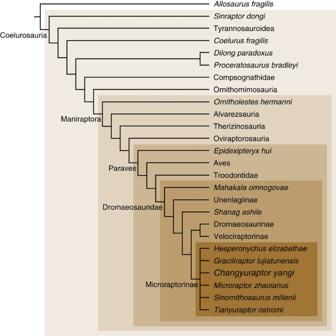Figure 5: Simplified strict consensus cladogram resultant from the phylogenetic analysis. The results of the analysis support the inclusion ofChangyuraptor yangiwithin microraptorine dromaeosaurids. Figure 5: Simplified strict consensus cladogram resultant from the phylogenetic analysis. The results of the analysis support the inclusion of Changyuraptor yangi within microraptorine dromaeosaurids. Full size image HG B016 can be assigned to Dromaeosauridae on the basis of the extremely elongate prezygapophyses and haemal arches that form bundles dorsal and ventral to the caudal vertebral centra, the presence of manual phalanx III-1 significantly longer (more than twice) than III-2, and a long metatarsal V. Comparisons to other dromaeosaurids indicate that HG B016 belongs to a new taxon, Changyuraptor yangi . Within dromaeosaurids, pennaceous feathers with a structure comparable to that of modern birds—shaft and barbs in a herringbone pattern—have only been documented for Microraptor zhaoianus [3] , [20] and Sinornithosaurus millenii [2] , [12] . In Sinornithosaurus millenii , these structures are relatively short, ~50 mm in the forelimb [12] . These structures are much better developed in Microraptor zhaoianus , in which the feathers of the forelimb and tail can reach up to 222 mm (primaries; IVPP V13352) and 185 mm (central pair of rectrices; IVPP V13351), respectively [3] . The rectrices of HG B016 are substantially longer than those of the largest known specimen of Microraptor zhaoianus , and they are even larger than the longest primaries of this species. Indeed, rectrices of Changyuraptor yangi ( Figs 2 and 4 ) constitute the longest feathers ever recorded in any non-avian theropod. Changyuraptor yangi is the second unquestionable dromaeosaurid (after Microraptor ) to possess ‘hindwings’, and by far the largest of all the known ‘four-winged’ dinosaurs. HG B016 is ~60% larger than IVPP V13352 (originally identified as the holotype of Microraptor gui [20] ) ( Table 1 ), which before discovery was the largest ‘four-winged’ dinosaur [3] . Small size has been previously noted as a potential key adaptation in microraptorines for aerial locomotion [3] , [18] , [23] , [24] . The morphology of Changyuraptor yangi suggests that aerial abilities (be it gliding, powered flight, incline running or other semi-aerial locomotion) were not necessarily limited to small-bodied animals but were also present among more sizable animals. The well-preserved and exceptionally long rectrices of HG B016 provide important information about the aerodynamic capabilities of the tail of microraptorines and may also help explain how large microraptorines could engage in some form of flight and/or controlled descents despite their size ( Supplementary Information ). The tail of microraptorines has been previously implicated as a pitch control structure [25] , [26] . Assuming that HG B016 is geometrically similar (that is, having the same proportions differing only in overall size) to IVPP V13352 provides a mass estimate of 4.0 kg for HG B016 (and therefore a weight of 39.2 newtons). Applying basic flat plate analysis for tail performance suggests that the lift generated by the tail fan of HG B016 could compensate for as much as 20% of its weight (in pitch) during small adjustments of the main wings. This result implies that the tail of Changyuraptor yangi and other microraptorines would be able to help compensate for small adjustments in pitch during aerial motion (gliding, powered flight or assisted leaps). Furthermore, the low aspect ratio of the tail of HG B016 ( Figs 2 and 4 ) would produce a relatively low ratio of lift to drag (L:D), which while reducing steady glide performance, could be highly adaptive for controlling rapid descent. It has been suggested that paravian dinosaurs may have used their lift surfaces to accomplish behaviours such as climbing inclines and controlling rapid descents from elevated perches [27] , [28] . Ultimately, it is the resultant force (total of lift and drag) that acts about the relevant moment arms to affect flight path. If the tail of HG B016 had a similar coefficient of drag to a high drag avian wing (CD of 0.13) [29] , then the L:D ratio for the tail would be barely greater than 1:1. As such, the angle of the resultant fluid force would be angled back from the oncoming air at ~45 degrees. This low L:D ratio force production would tend to reduce overall glide performance with regards to glide angle (that is, greater loss of height during shallow glides). However, it would provide some stabilization and a reduction of speed during steeper descents. These may have been important sources of stability and speed control in HG B016, especially since microraptorines likely lacked the forewing strength of modern birds. Combined with the possibility of passive flexion of the distal tail to take on both positive and negative angles of attack, this caudally oriented combination of lift and drag may have acted to reduce descent speed while simultaneously providing passive stability in the pitching axis, which could be critical to a safe landing or precise attack on prey. Such pitch stabilization could be particularly important for larger microraptorines (since they would tend to fly and/or descend more rapidly than small individuals), and this effect explains why the tail fan is exceptionally long in HG B016. A pitch control function also explains why the feathered tails of microraptorines are proportionally much longer than in other maniraptorans [30] , as this would extend the moment arm for pitch control by the tail. The discovery of HG B016 thus supports the hypothesis that the extended tail and long, fanned retrices of microraptorines played a key aerodynamic role, allowing them to retain aerial and/or semi-aerial competency at relatively large body sizes. The remarkably long-feathered tail Changyuraptor yangi helps us understand how such low-aspect-ratio tails operated as pitch control structures that reduced descent speed during landing. Authenticity of HG B016 The specimen was extensively prepared by staff (M. Walsh) of the Natural History Museum of Los Angeles County. Preparation revealed an attempt to artificially reconstruct the neck (see difference between photographs and composite line drawing in Fig. 1 ). The original cervical series is very poorly preserved. Nonetheless, remnants of the original cervical vertebrae as well as the contour of the neck feathering support the association of the skull and post-cranium, which clearly belong to the same animal and the same slab. The extensive preparation on the specimen supported that remaining portions of the skeleton and the plumage are authentic. Phylogenetic analysis The goal of this analysis was to test the phylogenetic placement of the new taxon Changyuraptor yangi within Paraves. The phylogenetic data set is from Turner et al . [19] and includes 109 species-level taxa, two generic-level taxa ( Unenlagia and Crax ) and 474 phenotypic characters. Turner et al . [19] provide detailed justification for use of genera for these two taxa. Our taxon-sampling scheme follows the primary analysis of Turner et al . [19] , with the exception that Pyroraptor olympius was excluded from the analysis. This does not affect the in-group topology of Dromaeosauridae, but it greatly reduces the number of most parsimonious trees. Characters 16, 17, 18, 27, 40, 68, 76, 110, 113, 125, 132, 157, 169, 174, 198, 200, 235, 265, 266, 269, 272, 284, 292, 314, 321, 324, 326, 331, 333, 356, 364, 369, 384, 390, 392, 398, 402, 406, 414, 418, 420, 422, 425, 430, 431, 432, 433, 438, 448 and 450 present potentially nested sets of homologies and/or entail presence and absence information. These characters were set as additive. Characters 6, 50 and 52 were excluded. The complete data set is available on Morphobank [31] at http://morphobank.org/permalink/?979 . The data set was analysed with equally weighted parsimony using TNT v. 1.0 (ref. 32 ). A heuristic tree search strategy was conducted performing 10,000 replicates of Wagner trees (using random addition sequences, RAS) followed by TBR branch swapping (holding 10 trees per replicate). The best trees obtained at the end of the replicates were subjected to a final round of TBR branch swapping. Zero-length branches [33] were collapsed if they lacked support under any of the most parsimonious reconstructions (that is, rule 1 of 35). This tree search strategy aims to obtain all the most parsimonious resolutions. The results of this search strategy produced 4,792 most parsimonious trees of 2,036 steps (CI=0.300, RI=0.740), found in 2,192 out of the 10,000 replications of RAS+TBR. Additional TBR branch swapping of these 2,192 trees found 10,096 additional optimal topologies, resulting in a total of 12,288 most parsimonious topologies. The strict consensus of the 12,288 most parsimonious trees is well resolved for Paraves, which relationships are the same as those found by Turner et al . [19] ( Fig. 5 ; Supplementary Fig. 4 ). Character support for the microraptorine node was calculated using two methods. The first is the jackknife applied to character resampling [34] . Farris et al . [34] and others [35] have given detailed reasons for preferring this measure over nonparametric bootstrap resampling [36] , which relies on assumptions not met by most morphological data sets. The second method used is Bremer support [37] , [38] , which evaluates node stability/sensitivity by examining suboptimal tree solutions to determine how many additional steps must be allowed in searching for topologies before the hypothesized clade is no longer recovered. Bremer support was calculated using negative constraints through the use of the BREMER.RUN script supplied with TNT. The jackknife analysis was calculated using TNT [32] using 1,000 replicates for which the probability of independent character removal was set to 0.20. Each jackknife replicate was analysed using a tree search strategy consisting of 10 replicates of RAS followed by TBR branch swapping (saving 10 trees per replicate). The topologies obtained during the jackknife replicates are summarized using GC frequencies. This follows the recommendations of Goloboff et al . [32] GC frequencies are preferable because they reflect the balance between the amounts of evidence that corroborates a given clade with the amount that falsifies that group. Support for the Microraptorinae node is low for both the Bremer and jackknife analyses. The node collapses in trees just one step longer and the GC frequency is only 3. Tail function equations and analysis Total lift for a simple wing at moderate to high Reynolds numbers can be calculated as: The coefficients of lift and drag are generally experimentally determined in living systems. This is obviously not possible for a fossil specimen. However, we can generate some boundaries for estimation. We observe that the tail fan of IVPP V13352 is not much more than a flat plate (perhaps with limited camber), and that it would operate at a low angle of attack during relatively level flight. For a thin plate at low angle of attack: where AR=aspect ratio (AR is, in turn, equal to b 2 / S where b =span and S is lifting surface area). Cl 0 , for a cambered plate at low angle of attack, is 2 π a, which yields: In this expression, ‘ a ’ is the angle of attack of the airfoil (relative to the airflow). If we assume that the tail fan of HG B016 performed roughly as good as a flat plate, we can therefore estimate the lift production as: To maintain pitch stability, the pitching moments generated by the tail and body would need to balance, such that: d (tail) is the distance of the tail fan from the centre of lift of the main wings, and d (cg) is the distance of the centre of gravity to the same point. We estimate the tail area as 0.041 m 2 and span of 0.12 metres. Air density is taken at sea level. At an angle of attack of 8° (0.14 radians) and air speed of 10 m s −1 , this yields 0.33 newtons of fluid force as lift. Assuming that the centre of lift sat near the elbow, this gives a d (tail) of ~0.63 metres, and a resultant moment of 0.207 newton metres. The amount of body weight producing a positive pitching moment that could be compensated by the tail would therefore be equal to ~0.207/ d (cg) newtons. As an example application of this expression, if the centre of lift from the main wings was moved 4 cm in front of the centre of mass, the tail (at an angle of attack of 8°) would compensate for ~8.0 newtons in pitch, which was ~20% of the total body weight of the animal. Nomenclatural acts This published work and the nomenclatural acts it contains have been registered in ZooBank, the proposed online registration system for the International Code of Zoological Nomenclature (ICZN). The ZooBank LSIDs (Life Science Identifiers) can be resolved and the associated information viewed through any standard web browser by appending the LSID to the prefix ‘ http://zoobank.org/ ’. The LSID for this publication is urn:lsid:zoobank.org:pub:BAC2D8C3-E572-4AEE-A277-F2928F32E5F6. How to cite this article: Han, G. et al . A new raptorial dinosaur with exceptionally long feathering provides insights into dromaeosaurid flight performance. Nat. Commun. 5:4382 doi: 10.1038/ncomms5382 (2014).